Interplay between phosphorylation and SUMOylation events determines CESTA protein fate in brassinosteroid signalling Brassinosteroids (BRs) are steroid hormones that are essential for plant growth. Responses to these hormones are mediated by transcription factors of the bri1 -EMS suppressor 1/brassinazole resistant 1 subfamily, and BRs activate these factors by impairing their inhibitory phosphorylation by GSK3/shaggy-like kinases. Here we show that BRs induce nuclear compartmentalization of CESTA (CES), a basic helix-loop-helix transcription factor that regulates BR responses, and reveal that this process is regulated by CES SUMOylation. We demonstrate that CES contains an extended SUMOylation motif, and that SUMOylation of this motif is antagonized by phosphorylation to control CES subnuclear localization. Moreover, we provide evidence that phosphorylation regulates CES transcriptional activity and protein turnover by the proteasome. A coordinated modification model is proposed in which, in a BR-deficient situation, CES is phosphorylated to activate target gene transcription and enable further posttranslational modification that controls CES protein stability and nuclear dynamics. Brassinosteroids (BRs) are steroid hormones of plants that control essential developmental programs [1] . The BRs are synthesized from the sterol campesterol, which is modified in a branched pathway to yield the bioactive BRs castasterone and brassinolide (BL) [2] . Castasterone and BL bioactivity is conferred by binding to the BR receptor BRI1 (brassinosteroid insensitive 1) [3] , which initiates a phosphorylation-dependent signal transduction cascade that leads to nuclear activation of transcription factors (TFs) that regulate BR responsive genes in their expression [4] , [5] , [6] . BES1 ( bri1 -EMS suppressor 1) and BZR1 (brassinazole resistant 1) are the best-studied BR-controlled transcriptional regulators of Arabidopsis thaliana (arabidopsis). They are substrates of arabidopsis GSK3/shaggy-like kinases (ASKs) such as BIN2 (brassinosteroid insensitive 2), which targets the proteins for phosphorylation to promote their degradation, restrict their cellular localization and inhibit their DNA-binding activity [5] , [6] . In addition to BES1 and BZR1, other TFs are also involved in regulating BR responses. These include a number of basic helix-loop-helix (bHLH) proteins, such as BEE1 (brassinosteroid-enhanced expression 1) to BEE3, which are induced by BRs [7] , BIM1 (BES1-interacting Myc-like 1) to BIM3 (ref. 8 ), which interact with BES1 in DNA binding, SPCH (speechless), which controls stomata development [9] and PIF4 (phytochrome-interacting factor 4), which interacts with BZR1 to integrate phytochrome signals into BR-regulated growth and development [10] , [11] . Another member of the bHLH TF family implicated in BR responses is CESTA (CES) [12] . CES is a homologue of BEE1 and BEE3 and regulates the expression of BR biosynthetic and other BR responsive genes [12] . CES is expressed in all organs and is enriched in floral and vascular tissues [12] , [13] . A loss of CES function results in shorter and only half-filled siliques [13] , whereas a gain of CES function promotes fertility and increases yields [13] , but also promotes elongation growth in other organs such as hypocotyls and leaves [12] . CES is a nuclear protein that heterodimerizes with BEE1 and can directly bind to G-box motifs in planta [12] . How CES activity is regulated has remained unknown, although we have shown previously that CES can be phosphorylated by BIN2 in vitro and that inhibition of ASK activity, by means of application of bikinin [14] , induces CES compartmentalization in nuclear bodies (NBs) [12] . NBs are subnuclear foci of different kinds to which a number of plant proteins localize [15] . These include multiple factors involved in light signalling such as the red/far-red light receptors phytochromes (PHYs) A and B and the bHLH proteins phytochrome-interacting factors PIF3, PIF7 and HFR1 (long hypocotyl in far-red 1), all of which associate with phytochrome NBs in a light-responsive manner [16] . However, to date NB formation has not been implicated in BR signalling, and the modes which enable subnuclear dynamics of plant proteins have remained elusive. In this work, we carried out a mutational analysis of CES to define the structural requirements for BR-induced NB localization and identify an extended SUMOylation motif, in which phosphorylation antagonizes SUMOylation. We show that interfering with SUMOylation inhibits NB association and that promoting SUMOylation induces constitutive nuclear compartmentalization, revealing that SUMOylation controls CES NB localization. Moreover, we identify a main BIN2 target site and provide evidence that phosphorylation controls CES activity and protein stability. A model is proposed in which, in a BR-deficient situation, CES is phosphorylated by BIN2 to increase CES transcriptional activity on specified target promoters. In response to an activation of BR signalling, CES undergoes further posttranslational modification to alter CES activity and determine CES protein fate. SUMOylation controls CES NB localization CES nuclear re-localization in response to BRs is detectable only when a pre-treatment with the BR biosynthesis inhibitor brassinazole (Brz) [17] is performed [12] . This indicated that a BR-deficient state may promote CES nuclear compartmentalization [12] . To test this hypothesis, we introduced a 35S:CES wt -YFP reporter [12] into the BR-deficient mutant background cpd (constitutive photomorphogenesis and dwarfism) [18] by crossing and analysed CES wt -YFP nuclear re-localization in the progeny. As shown in Fig. 1a , in the cpd background, CES wt -YFP localized diffusely in the nucleus in untreated conditions. However, when seedlings were treated with BL for 2 h, CES wt -YFP re-localization to NBs was evident without a Brz pre-treatment ( Fig. 1a ). This re-localization occurred in a tissue-specific manner, being prominent in particular in vascular tissues and stomata, was rapid and was reverted equally fast underscoring the highly dynamic nature of this process. 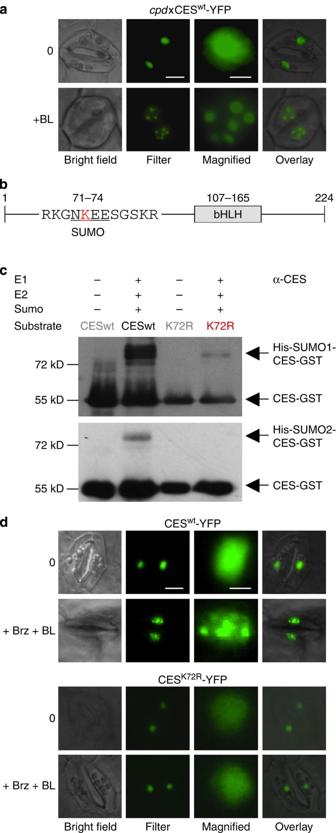Figure 1: K72 is a SUMOylation site that controls BR-induced CES nuclear body localization. (a) Fluorescence microscopic images of representative stomata of 14-day-oldcpd x 35S:CESwt-YFP/32seedlings either untreated (upper panel) or treated with 1 μM BL for 2 h (lower panel). Scale bars: filter, 5 μm, magnified, 2 μm. (b) Structure of the CES protein with the SUMOylation motif underlined. Target lysine in red. (c)In vitroSUMOylation assays using the heterodimeric SUMO-activating enzyme E1 and SUMO-conjugating enzyme E2, SUM1 and SUM2 as modifiers, and assessing affinity purified, recombinant GST-CESwtand GST-CESK72Ras substrate proteins. (d) Representative fluorescence microscopic images of stomata of 14-day-old plants of35S:CESwt-YFP(line 32, upper two rows) or35S:CESK72R-YFP(line 411, lower two rows) either untreated (upper row) or treated with 1 μM Brz for 24 h followed by 1 μM BL for 2 h (lower row). Figure 1: K72 is a SUMOylation site that controls BR-induced CES nuclear body localization. ( a ) Fluorescence microscopic images of representative stomata of 14-day-old cpd x 35S:CES wt -YFP/32 seedlings either untreated (upper panel) or treated with 1 μM BL for 2 h (lower panel). Scale bars: filter, 5 μm, magnified, 2 μm. ( b ) Structure of the CES protein with the SUMOylation motif underlined. Target lysine in red. ( c ) In vitro SUMOylation assays using the heterodimeric SUMO-activating enzyme E1 and SUMO-conjugating enzyme E2, SUM1 and SUM2 as modifiers, and assessing affinity purified, recombinant GST-CES wt and GST-CES K72R as substrate proteins. ( d ) Representative fluorescence microscopic images of stomata of 14-day-old plants of 35S:CES wt -YFP (line 32, upper two rows) or 35S:CES K72R -YFP (line 411, lower two rows) either untreated (upper row) or treated with 1 μM Brz for 24 h followed by 1 μM BL for 2 h (lower row). Full size image In mammalian cells, conjugation of proteins with small ubiquitin-like modifiers (SUMO) plays a central role in nuclear compartmentalization [19] , [20] . Therefore, we analysed the CES sequence utilizing the SUMOsp 2.0 software [21] and identified a motif, 71-NKEE-74 ( Fig. 1b ), which bears analogies with the SUMOylation consensus ΨKX(E/D) [22] . To assess if CES is SUMOylated and whether lysine (K) 72 may be a target, K72 was mutated to arginine (R) and both mutant and wild-type CES were purified as GST fusion proteins from Escherichia coli . In vitro SUMOylation assays were then carried out with the SUMO isoforms SUM1 or SUM2 as modifiers and CES wt -GST or CES K72R -GST as substrates, detecting CES products by western blotting with an α-CES peptide antibody. The results showed that CES was SUMOylated by both SUM1 and SUM2 in vitro and, importantly, that K72R strongly reduced SUMOylation of CES with SUM1 and abolished SUMOylation with SUM2 ( Fig. 1c ). To investigate the in planta consequences of interfering with CES SUMOylation, plants stably overexpressing CES K72R -YFP were generated. We decided to deliver all CES variants generated in this work ectopically, utilizing the constitutive 35S promoter rather than the endogenous CES promoter, which is active in specific tissues only [12] . This approach was chosen to facilitate detection of SUMOylated CES in vivo , since SUMOylated protein states are generally transient and highly unstable. Moreover, only a small fraction is typically SUMOylated in vivo , making the biochemical detection very challenging [23] . Two independent CES K72R -YFP -expressing lines with comparable CES mRNA levels as two CES wt -YFP -expressing controls were selected by quantitative PCR (qPCR) ( Supplementary Fig. 1 ). When CES-YFP nuclear localization was studied in these lines, it was found that, in analogy to CES wt , the CES K72R mutant localized diffusely in the nucleus in non-induced conditions ( Fig. 1d ). However, importantly, when CES K72R -YFP plants pre-treated with Brz were treated with BL, unlike CES wt , CES K72R did not re-localize to NBs, showing that the SUMO target site K72 is required for CES NB localization ( Fig. 1d ). Phosphorylation antagonizes CES SUMOylation in planta K72 is in close proximity to two putative phosphorylation sites: serines (S) 75 and 77. Since phosphorylation near SUMO attachment sites can alter SUMOylation in animal systems [22] , [24] , we hypothesized that phosphorylation of S75 and/or S77 could affect CES SUMOylation. To test this, a double mutant mutated in both sites (to alanines, A) was constructed, GST fusion proteins of CES wt and CES S75A+S77A were purified from E. coli , and in vitro kinase assays were carried out with protein extract of floral tissues in which CES is highly expressed [12] , [13] . The result showed that phosphorylation of the mutant was strongly reduced as compared with wild-type ( Fig. 2a ), providing evidence that S75 and/or S77 are in vivo phosphorylation sites. 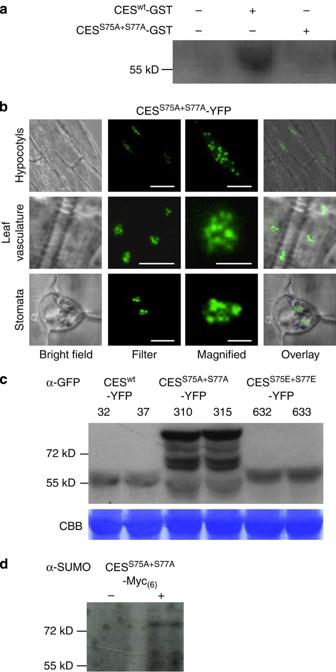Figure 2: Mutating serine 75 and 77 to alanine promotes SUMOylation and increases CES protein stability. (a)In vitrokinase assays with affinity purified recombinant CESwt-GST or CESS75A+S77A-GST protein, [γ-32P]ATP and total plant extracts fromArabidopsisflowers. (b) Confocal microscopic images showing CESS75A+S77A-YFP localization in different tissues of 2-week-old plants. Scale bars: hypocotyls: filter, 40 μm, magnified, 5 μm; leave vasculature: filter, 40 μm, magnified, 5 μm; stomata: filter, 5 μm, magnified, 2 μm. (c) Immunoblotting of protein extracts of 2-week-old seedlings of the indicated lines using α-GFP antibody for CES-YFP detection. Upper panel: autoradiogram, lower panel: coomassie brilliant blue staining (CBB) as a loading control. (d) Detection of SUMOylated CESin vivo. CES was immuno-precipitated fromArabidopsisprotoplasts transiently expressing35S:CESS75A&S77A-Myc(6)(please note that CES tagged withMyc(6)is smaller as compared with CES tagged with YFP) using α-Myc antibody and detected by immunoblotting with an α-SUMO antibody. Figure 2: Mutating serine 75 and 77 to alanine promotes SUMOylation and increases CES protein stability. ( a ) In vitro kinase assays with affinity purified recombinant CES wt -GST or CES S75A+S77A -GST protein, [γ- 32 P]ATP and total plant extracts from Arabidopsis flowers. ( b ) Confocal microscopic images showing CES S75A+S77A -YFP localization in different tissues of 2-week-old plants. Scale bars: hypocotyls: filter, 40 μm, magnified, 5 μm; leave vasculature: filter, 40 μm, magnified, 5 μm; stomata: filter, 5 μm, magnified, 2 μm. ( c ) Immunoblotting of protein extracts of 2-week-old seedlings of the indicated lines using α-GFP antibody for CES-YFP detection. Upper panel: autoradiogram, lower panel: coomassie brilliant blue staining (CBB) as a loading control. ( d ) Detection of SUMOylated CES in vivo . CES was immuno-precipitated from Arabidopsis protoplasts transiently expressing 35S:CES S75A&S77A -Myc (6) (please note that CES tagged with Myc (6) is smaller as compared with CES tagged with YFP) using α-Myc antibody and detected by immunoblotting with an α-SUMO antibody. Full size image To test the hypothesis that phosphorylation of S75 and/or S77 impacts on CES SUMOylation also, a mutant was generated in which S75+S77 were replaced by glutamic acid (E) to mimic constitutive phosphorylation. YFP-fusion proteins were generated with both double mutants, and lines with comparable transgene expression were identified using qPCR ( Supplementary Fig. 1 ). When CES-YFP localization was studied, it was found that CES S75E+S77E behaved like CES wt (showing subnuclear re-localization in response to BR, Supplementary Fig. 2a ), whereas the CES S75A+S77A mutant localized constitutively to subnuclear compartments in different tissues, including the vasculature of roots and the hypocotyl and in stomata ( Fig. 2b ). Importantly, although the CES S75A+S77A mutant was delivered ectopically, constitutive ‘speckling’ was not detectable in all tissues, but was seen particularly in cell types where CES is naturally most abundant, including stomata and vascular tissues [12] , and where also CES wt -YFP speckles BR-induced, indicating cell type specificity of the components that control CES NB localization. To study the impact of mutating S75 and S77 on CES protein fate, western blots were performed. In CES wt -YFP - and CES S75E+S77E -YFP -expressing lines bands with a molecular mass of ~53 kD (the expected CES-YFP size) were detected. On the contrary in CES S75A+S77A -YFP plants, a number of stronger bands with higher molecular weight appeared ( Fig. 2c ). To test whether the larger molecular weight bands in CES S75A+S77A -YFP plants are SUMOylated protein states, a 35S:CES S75A+S77A -Myc (6) construct was expressed in Arabidopsis protoplasts, the fusion protein was immuno-precipitated using an α-Myc antibody and a western blot with α-SUMO antibody was performed. The result showed that CES S75A+S77A - Myc (6) was SUMOylated in vivo ( Fig. 2d ). Since CES S75A and S77A single mutations did not impact on CES nuclear localization ( Supplementary Fig. 2b ) or protein size in planta ( Supplementary Fig. 2c ), there is evidence that phosphorylation of one site only is sufficient to antagonize SUMOylation. Plant lines overexpressing CES wt -YFP also infrequently showed higher molecular weight bands ( Supplementary Fig. 2d ). However, these bands were very faint reflecting that, like other SUMOylated proteins [23] , only a small CES fraction is naturally SUMOylated. Moreover, the result gives support to the notion that SUMOylated CES protein states are highly unstable, being stabilized only when phosphorylation at S75 and S77 is prevented. T35 controls CES protein abundance We have shown previously that BIN2 can phosphorylate CES in vitro [12] . Moreover, bikinin can induce CES nuclear compartmentalization [12] , suggesting that ASK-mediated phosphorylation regulates CES protein fate. In support, in the bin2-1 mutant background where BIN2 is constitutively active [25] , CES-YFP re-localizes to NB only in response to bikinin, but not to BL ( Supplementary Fig. 2e ), providing evidence that CES NB localization is under ASK control. To investigate if ASKs can directly interact with CES, in vivo bimolecular fluorescence complementation assays [26] were carried out in Arabidopsis protoplasts. For this purpose, ASKθ was chosen, since it is expressed to reasonable levels in protoplasts (whereas BIN2 is weakly expressed in this system [27] ). When ASKθ and CES, fused to the C-terminal and N-terminal portions of YFP, respectively, were co-expressed in protoplasts, yellow fluorescence was seen ( Supplementary Fig. 3a ). Therefore, there was evidence that ASKθ can interact with CES in vivo . Since CES does not contain a classical GSK3 recognition motif (S/TxxxS/T P in tandem repeats) [28] , a mass spectrometric analysis of BIN2-phosphorylated CES was performed, which revealed four amino-acid residues, T35, T95, S116 and S182, to be phosphorylated in vitro . Contrary to our expectations, BIN2 did not phosphorylate S75 or S77. Site-directed mutagenesis and subsequent in vitro kinase assays, employing single mutants (substitutions to A), revealed that CES T35A strongly impaired BIN2-mediated phosphorylation ( Fig. 3a ). A quadruple mutant (CES T35A+T95A+S116A+S182A ) exhibited a comparable reduction in phosphorylation as the CES T35A single mutant showing that T35 is the primary amino acid required for BIN2 phosphorylation in vitro . 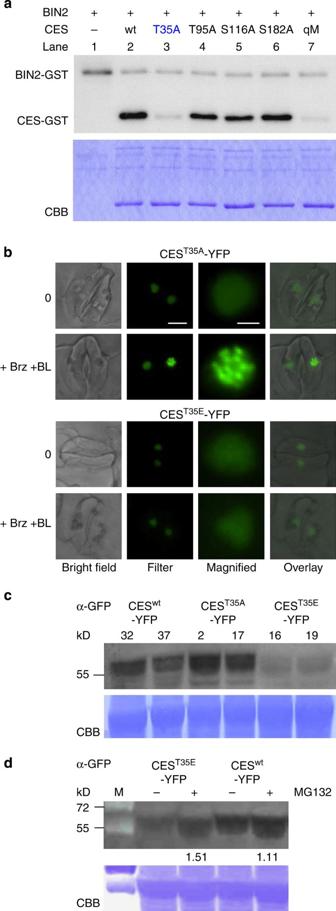Figure 3: T35 is a BIN2 target site that controls CES protein stability. (a)In vitrokinase assays using recombinant BIN2-GST and different GST-tagged CES variants; qM (quadruple mutant). CBB staining is shown as a loading control. (b) Representative fluorescence microscopic images of stomata of 14-day-old plants of 35S:CEST35A-YFP (line 2, upper two rows) or 35S:CEST35E-YFP (line 19, lower two rows) either untreated (upper rows) or treated for 24 h with 1 μM Brz followed by 2 h of 1 μM BL (lower rows). Scale bars: filter, 5 μm, magnified, 2 μm. (c) Immunoblotting of protein extracts of 2-week-old seedlings of the indicated lines using α-GFP antibody for CES-YFP detection. Upper panel: autoradiogram, lower panel: coomassie brilliant blue staining (CBB) as a loading control. (d) Immunoblotting of protein extracts of 7-day-old seedlings of35S:CEST35E-YFP/16and35S:CESwt-YFP/32in the presence or absence of MG132 (3-h treatment) using α-GFP antibody for CES-YFP detection. Bands were quantified with the image-quant software and the increase as compared to the untreated control was calculated. CBB staining is shown as a loading control. Figure 3: T35 is a BIN2 target site that controls CES protein stability. ( a ) In vitro kinase assays using recombinant BIN2-GST and different GST-tagged CES variants; qM (quadruple mutant). CBB staining is shown as a loading control. ( b ) Representative fluorescence microscopic images of stomata of 14-day-old plants of 35S:CES T35A -YFP (line 2, upper two rows) or 35S:CES T35E -YFP (line 19, lower two rows) either untreated (upper rows) or treated for 24 h with 1 μM Brz followed by 2 h of 1 μM BL (lower rows). Scale bars: filter, 5 μm, magnified, 2 μm. ( c ) Immunoblotting of protein extracts of 2-week-old seedlings of the indicated lines using α-GFP antibody for CES-YFP detection. Upper panel: autoradiogram, lower panel: coomassie brilliant blue staining (CBB) as a loading control. ( d ) Immunoblotting of protein extracts of 7-day-old seedlings of 35S:CES T35E -YFP/16 and 35S:CES wt -YFP/32 in the presence or absence of MG132 (3-h treatment) using α-GFP antibody for CES-YFP detection. Bands were quantified with the image-quant software and the increase as compared to the untreated control was calculated. CBB staining is shown as a loading control. Full size image We mutated T35 to E, to also generate a phospho-mimeic version, stably expressed both mutants as YFP-fusion proteins in plants and selected lines with comparable transgene expression by qPCR ( Supplementary Fig. 1 ). When BR-induced nuclear re-localization was assessed in CES T35A - and CES T35E -expressing plants, it was found that whereas CES T35A re-localized to NB very efficiently, the CES T35E variant was compromised in this ability ( Fig. 3b ). In addition, the T35E mutation also had an effect on CES protein abundance. Protein immunoblotting revealed that, whereas CES T35A was present in comparable amounts like CES wild type in the transgenic lines, protein levels of CES T35E were clearly reduced ( Fig. 3c ). To assess if CES may be subjected to proteasomal degradation and if T35 phosphorylation may play a role, seedlings of 35S:CES wt -YFP were treated with the proteasome inhibitor MG132 and protein levels were determined by western blot analysis. The result showed that MG132 increased CES protein abundance ( Supplementary Fig. 4a ) and did so in a time-course manner following treatment ( Supplementary Fig. 4b ). To investigate if T35E may facilitate proteasomal degradation, CES T35E -expressing plants were treated with MG132 and protein abundance was assessed. As shown in Fig. 3d (and in Supplementary Fig. 4c with further biological replicates), after 3 h of MG132 treatment, CES T35E protein levels markedly increased providing evidence that T35E promotes CES degradation by the 26S proteasome. CDPKs phosphorylate CES within the extended SUMO motif Since S75 and S77 are not BIN2 target sites, we aimed to identify kinases that can catalyse S75 and S77 phosphorylation. We manually inspected the motif in which S75 and S77 are positioned and noted that it is flanked by basic and acidic polar residues, which form a repeat of two classical calcium-dependent protein kinase (CDPK) phosphorylation sites (‘simple 1’: basic-X-X-S/T and ‘simple 2’: S-X-R [29] ; Fig. 4a ). To assess if S75 and S77 may be targeted by CDPKs for phosphorylation in planta , we treated CES wt -YFP -expressing plants with trifluoperazine dihydrochloride (TFP), which inhibits plant CDPK activity [30] . CES wt -YFP localization was used as readout for accumulation of CES de-phosphorylated at S75 and S77. The result showed that TFP treatment induced nuclear compartmentalization of CES wt -YFP ( Fig. 4b ). Importantly, unlike CES wt -YFP, CES S75E+S77E -YFP did not re-localize to NB in response to TFP treatment ( Fig. 4b ) providing support that TFP induces de-phosphorylation of CES at S75 and S77 in planta . 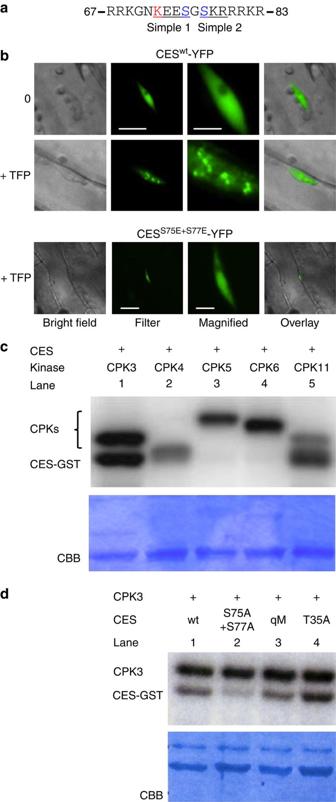Figure 4: CDPKs phosphorylate CES. (a) Sequence of the extended SUMOylation motif. The simple 1 (basic-XX-S/T) and simple 2 (S-X-R) CDPK recognition sites are underlined. K72 in red, S75 and S77 in blue. (b) Fluorescence microscopic images of hypocotyls of 14-day-old seedlings of35S:CESwt-YFP/32(upper panel) or35S:CESS75E+S77E-YFP/632 (lower panel), untreated or treated with 300 μM triflouperazine (TFP) for 1.5 h. Scale bars:CESwt-YFP: filter, 20 μm, magnified, 5 μm;CESS75E+S77E-YFP: filter, 20 μm, magnified, 5 μm. (c)In vitrokinase assays using recombinant, GST-tagged CES and CPK3, CPK4, CPK5, CPK6 and CPK11. CBB staining is shown as a loading control. (d)In vitrokinase assays with CPK3 using recombinant, GST-tagged CES mutant variants. CBB staining is shown as a loading control. Figure 4: CDPKs phosphorylate CES. ( a ) Sequence of the extended SUMOylation motif. The simple 1 (basic-XX-S/T) and simple 2 (S-X-R) CDPK recognition sites are underlined. K72 in red, S75 and S77 in blue. ( b ) Fluorescence microscopic images of hypocotyls of 14-day-old seedlings of 35S:CES wt -YFP/32 (upper panel) or 35S:CES S75E+S77E -YFP /632 (lower panel), untreated or treated with 300 μM triflouperazine (TFP) for 1.5 h. Scale bars: CES wt -YFP : filter, 20 μm, magnified, 5 μm; CES S75E+S77E -YFP : filter, 20 μm, magnified, 5 μm. ( c ) In vitro kinase assays using recombinant, GST-tagged CES and CPK3, CPK4, CPK5, CPK6 and CPK11. CBB staining is shown as a loading control. ( d ) In vitro kinase assays with CPK3 using recombinant, GST-tagged CES mutant variants. CBB staining is shown as a loading control. Full size image To investigate if CDPKs can directly phosphorylate CES, in vitro kinase assays were carried out. We picked five different CDPKs for this analysis: CPK3, a member of the CDPK subfamily II and CPK4, 5, 6 and 11, members of subfamily I [31] . Interestingly, CES was phosphorylated by CPK3 and CPK11, whereas CPK4, 5 and 6 did phosphorylate CES in vitro ( Fig. 4c ). To assess if CES may be phosphorylated at S75 and S77, the kinase assays were repeated to compare wild-type CES with CES S75A+S77A , the qM (CES T35A+T95A+S116A+S182A ) and CES T35A as substrates of CPK3. The result, shown in Fig. 4d , illustrates that CES wt , CES T35A and the qM were efficiently phosphorylated, whereas the phosphorylation activity of CPK3 against CES S75A+S77A was reduced, showing the CPK3 can phosphorylate CES at S75 and S77. To test if CPK3 and CPK11 physically interact with CES in planta , bimolecular fluorescence complementation assays were carried out. A fluorescence signal was observed both when protoplasts were co-transformed with split-YFP constructs of CPK3 and CES or CPK11 and CES ( Supplementary Fig. 2b ). Therefore, there is evidence that CPK3 and CPK11 can interact with CES in vivo . Phosphorylation and SUMOylation regulate CES activity To assess if altering phosphorylation and/or SUMOylation impacts on CES transcriptional activity, we performed luciferase (LUC) reporter transactivation assays in Arabidopsis protoplasts utilizing the Ren -Luc system [32] . A LUC reporter was cloned, in which LUC expression is driven by the promoter of CYP718 , a direct CES target in planta [12] . This reporter was co-expressed with wild-type CES or the different CES mutant variants in protoplasts generated from the haf bee1 bee3 mutant, a triple mutant deficient in the expression of CES/HAF and BEE1 and BEE3 (ref. 13 ) and LUC activity was assessed. The results showed that the K72R SUMO-deficient mutation reduced CES transcriptional activity on the CYP718 promoter, whereas the S75A+S77A mutations, which promote CES SUMOylation in planta , also increased CES activity ( Fig. 5a ). Also the phospho-mimeic S75E+S77E mutant was impaired in inducing pCYP718:LUC -reporter transcription. Interestingly, the T35 mutants behaved differently: T35A abolished CES transcriptional activity and also the T35E phospho-mimeic mutation reduced the transactivation activity of CES in this assay to some extent ( Fig. 5a ) showing that both modifications of T35 impacted on CES activity in this assay. 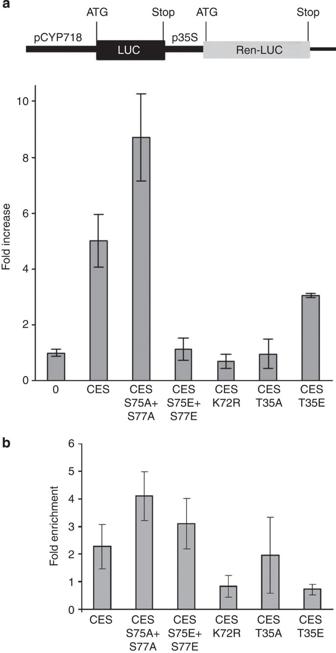Figure 5: Phosphorylation regulates CES activity. (a) The LUC reporter construct shown was transiently expressed in protoplasts generated fromhaf bee1 bee3plants either alone (0) or with the effectors CES, CESS75A+S77A, CESS75E+S77E, CESK72R, CEST35Aor CEST35E. Theyaxis is fold increase in the ratio between the activities of firefly LUC (under control of theCYP718promoter) and 35S promoter-driven controlRenillaLUC (Ren-LUC). The s.d. of three independent biological replicates is shown. (b) Chromatin-immunoprecipitation (ChIP) experiments with different plants expressing wild-type or mutant CES-YFP reporter lines using an α-GFP antibody for CES-YFP precipitation. The enrichment of a G-box containing fragment of theCPDpromoter in the antibody containing fraction (as compared with the control without antibody) was quantified by real-time PCR from immuno-precipitated samples. The s.d. of three biological replicates is shown. Figure 5: Phosphorylation regulates CES activity. ( a ) The LUC reporter construct shown was transiently expressed in protoplasts generated from haf bee1 bee3 plants either alone (0) or with the effectors CES, CES S75A+S77A , CES S75E+S77E , CES K72R , CES T35A or CES T35E . The y axis is fold increase in the ratio between the activities of firefly LUC (under control of the CYP718 promoter) and 35S promoter-driven control Renilla LUC ( Ren -LUC). The s.d. of three independent biological replicates is shown. ( b ) Chromatin-immunoprecipitation (ChIP) experiments with different plants expressing wild-type or mutant CES-YFP reporter lines using an α-GFP antibody for CES-YFP precipitation. The enrichment of a G-box containing fragment of the CPD promoter in the antibody containing fraction (as compared with the control without antibody) was quantified by real-time PCR from immuno-precipitated samples. The s.d. of three biological replicates is shown. Full size image In order to assess CES DNA-binding capacities to in vivo targets, we performed chromatin-immunoprecipitation experiments in which CES DNA-binding capacities to the promoter of the BR biosynthesis gene CPD , another known direct CES target [12] , were investigated. The result is given in Fig. 5b and shows that with CES S75A+S77A an increased enrichment, as compared with CES wt , was detected, whereas with the CES K72R and CES T35E mutants enrichment was reduced. These results correlated with the transactivation assays and for CES S75A+S77A and CES T35E also with the protein abundance in the transgenic lines. The CES S75E+S77E and CES T35A mutants did not show significantly altered enrichment as compared with CES wt , indicating that the reduced transactivation abilities do not stem from a reduced DNA-binding capacity of the mutants. BRs are steroid hormones of plants, which control multiple stages of plant growth and development. At present, it is understood that this ability is conferred by the activity of ASKs such as BIN2 that in the absence of BRs are activated to phosphorylate TFs of the BES1/BZR1 family, which reduces their activity and promotes their degradation by the proteasome [11] , [33] . Here we provide evidence for an expanded regulatory repertoire of BR signalling, which controls the activity of the TF CES as well as its protein stability and subnuclear dynamics, evidenced by an accumulation in NBs in response to BRs. NBs are dynamic, self-organizing structures whose structural integrity is mediated by transient protein–protein and likely protein–RNA interactions [19] . NBs are formed to govern specific activities associated with gene expression and genome maintenance, and are implicated in key cellular functions [19] . In plants, NB assembly is an early and essential event in light signalling with a variety of signalling components, including certain PIFs, localizing to NBs in a light-responsive manner by presently unknown means [16] , [34] . In this work, we show for the first time that SUMOylation can regulate NB formation in plants. A SUMOylation-impaired mutant was defective in re-localizing to subnuclear compartments, whereas a constitutively SUMOylated variant constitutively localized to subnuclear foci, demonstrating a direct role of SUMOylation in CES NB formation. Interestingly, previously there were indications that SUMOylation participates in NB localization of plant proteins. LAF1 (long after far-red light 1), a MYB TF that functions in PHYA signalling, was defective in nuclear compartmentalization when a mutation in an atypical SUMOylation motif was introduced [35] . Therefore, it is possible that like in animal systems [19] , [20] , SUMO may serve as an earmark to target multiple protein substrates to NBs in plants. In addition to showing that CES is SUMOylated, we provide evidence that it is a target of phosphorylation and that these posttranslational modifications cross-talk in the control of CES protein activity and fate. In plants, this is the first report to show that phosphorylation regulates SUMOylation and we identify a novel extended SUMOylation motif in which phosphorylation of serines 75 and 77 antagonizes SUMOylation at K72. Phosphorylation in the extension of SUMOylation motifs is known to control SUMOylation in animal systems; however, to date in all published cases, phosphorylation of such motifs was found to increase SUMOylation and in many cases convert TFs from activators to repressors [22] . This is not the case for CES since abolishing phosphorylation at serines 75+77 promotes SUMOylation and increases CES transcriptional activity. Also, the SUMOylation-impaired CES K72R mutant is less active in DNA binding, arguing against a model in which SUMOylation is a general means of compromising CES activity. Since SUMOylation induces CES NB assembly, it is possible that in NBs, conditional protein–protein interactions are favoured, which promote activity on certain promoters and restrict activity on others. This would allow for BRs to realize the suspected dual role of CES as both activator and repressor of gene expression [4] depending on the requirements and would be in analogy to the dual activities of BES1 and BZR1 (ref. 4 ). Since constitutively SUMOylated CES S75A+S77A accumulates to elevated levels in planta , it is conceivable that SUMOylation stabilizes the protein for example, by antagonizing ubiquitination, a role of SUMOylation in animal cells [22] , [24] . However, it is also possible that elevated CES levels are not the consequence of, but the cause for SUMOylation. A role in proteolysis was recently postulated for PHY-containing NBs, since plants defective in PHY NB assembly are also impaired in PHYA, PIF1 and PIF3 degradation [36] , [37] . In this context, it is interesting to note that CES does not co-localize with COP1 (constitutive photomorphogenis 1, Supplementary Fig. 5 ), a marker for PHY-containing NB [38] , [39] , indicating that CES localizes to a different NB class and this will be addressed in future work. The fact that serines 75 and 77 are part of two classical CDPK recognition sites allowed us to identify CDPKs as candidates for catalysing CES phosphorylation within the extended SUMOylation motif. We show that CPK3 and CPK11 can interact with CES in vivo , can phosphorylate CES in vitro and that S75 and S77 are CPK3 target sites. Moreover, TFP, an inhibitor of CDPKs [30] , induces CES NB formation providing first evidence for a potential role of CDPKs in phosphorylating CES in planta and this will have to be verified. Importantly, CES is also phosphorylated by BIN2 (ref. 12 ) and here we provide in vitro evidence that T35, which is not part of a classical GSK3 phosphorylation motif, is required for BIN2 phosphorylation. In animal systems, GSK3/shaggy-like kinases can phosphorylate a consensus typically composed of tandem repeats of (S/TxxxS/T P ) where the second S/T is often the site of a priming phosphorylation [28] . However, in addition, GSK3 substrates exist that lack a putative priming site [28] , [40] . In plants, only one study has been published today where an in vivo target sites of a GSK3 has been identified [41] . It is glucose-6-dehydrogenase that is phosphorylated by ASKα at Thr-467 (ref. 41 ), which is also not part of a classical GSK3 motif. In many other cases, evidence exists that proteins are phosphorylated by GSK3s; however, the in vivo phosphorylation sites have not been determined. These include BES1 and BZR1 that are phosphorylated by ASKs in planta [42] ; however, the in vivo phosphorylation sites remain unknown. Clearly, it will be important to determine which ASKs can phosphorylate CES in planta and if T35 is a target for ASK phosphorylation. Phosphorylation of T35 regulates CES protein stability, and we provide evidence that it serves as a tag to mark CES for proteasomal degradation. In addition, our results suggest that T35 phosphorylation can enhance CES transcriptional activity, since mutation of T35 reduces CES transactivation abilities. This is in contrast to the proposed regulatory role of BIN2-mediated phosphorylation in BES1/BZR1 activity, which is thought to constitute an inactivation reaction [33] , [43] . Therefore, our results suggest a novel concept of BR signalling in which, in a BR-depleted situation, ASKs phosphorylate CES at T35 to increase CES activity on selected promoters. This could be utilized to enhance CES activity on promoters that must be activated when BR levels are low such as BR biosynthesis genes. Indeed, it is known that BR biosynthetic gene expression rapidly increases when BRs are depleted [44] and here we provide the first molecular explanation how this feedback induction may function. Since mimicking phosphorylation at T35 also promotes protein turnover, in our model, active CES, earmarked at T35, would be degraded by the proteasome. In response to BRs, active CES would be rapidly moved to NBs. Moreover, newly translated CES would accumulate in a T35 non-phosphorylated form, which would facilitate phosphorylation at S75+S77 to retain CES inactive on specific promoters. Since CES NBs are very transient structures, it is possible that CES is de-sumoylated when BR levels become low. It is also possible that SUMOylation serves as a tag for subsequent processing in NBs such as ubiquitination and degradation and this will have to be determined. In plants, little is known yet about the regulatory roles of SUMOylation. The identification of SUMOylation of CES is an essential first step in understanding the significance of SUMOylation in the nuclear processing and compartmentalization of BR-regulated TFs and provides a foundation for elucidating its contribution to the regulation of BR responsive growth and development in the future. Plant material and growth conditions Arabidopsis thaliana Colombia-0 was the ecotype used in this study. All mutants and transgenic lines generated are in this background. For plant propagation, seeds were sterilized using the chlorine vapour method [45] and plated on half strength Murashige and Skoog (½ MS) medium [46] . After stratification at 4 °C for 2 days, plates were placed in a growth chamber at 21±2 °C and usually incubated vertically in long-day growth conditions (16 h of 80 μmol m −2 s −1 cool white light/8 h dark). Treatments were generally performed with plants transferred to liquid ½ MS media, which were then adapted to growth in liquid medium for 24 h before chemicals were applied. Molecular cloning and generation of transgenic Arabidopsis CES mutants were generated by site-directed mutagenesis using the primer pairs given in Supplementary Table 1 . Obtained PCR products were cloned Nco I +Not I into the binary plant expression vector pGWR8 (ref. 47 ) downstream of the CaMV35S promoter. For generation of YFP-fusion constructs or Myc -tagged version, the YFP-tag or 6x Myc -tag was added in frame as a Not I fragment to the C-terminal parts of CES mutants. Plants were transformed with the constructs using the floral dip method [45] and at least 10 independent transgenic lines were selected for each construct for further analysis. For co-localization experiments, the coding sequence of COP1 was PCR amplified from Arabidosis cDNA and the PCR product was cloned as Nco I +Not I fragment into the binary plant expression vector pGWR8 (ref. 47 ) downstream of the CaMV35S promoter. The CFP tag was added in frame as a Not I fragment to the C-terminal part of COP1. For recombinant protein production, CES or CES mutants were cloned Nco I +Not I in frame with the GST coding sequence into pGEX-4T2 (GE Healthcare, Buckinghamshire, UK). For cloning of the pCYP718:LUC construct, a 3.3-kb fragment of the CYP718 promoter upstream from the translational start was PCR amplified from genomic DNA using specific primers and cloned Not I +Nco I into the pGreen008-II-Luc vector [32] in frame with the coding sequence of the LUC gene. For in vitro SUMOylation assays, the plasmids from ref. 48 were modified. The pCDFDeut-AtSUMO1/2-AtSCE1 plasmids were digested with Xho I+ Sal I to remove the AtSCE1 coding sequence and the plasmid backbone was then self-ligated. This resulted in a plasmid containing the coding sequence for mature SUMO isoforms (with exposed C-terminal di-Glycine motif) in frame with a N-terminal HIS-tag. For in vitro kinase assays with CDPKs, AtCPK3, AtCPK4, AtCPK5, AtCPK6 and AtCPK11 were amplified from Arabidopsis cDNA using the primer pairs given in Supplementary Table 1 and were cloned into the pTWIN1 vector (New England Biolabs, Ipswich, MA, USA) in frame with an intein-tag. YFP localization studies For YFP localization studies, transgenic seedlings expressing CES S75A+S77A -YFP were grown on ½ MS plates for 11 days and subsequently analysed with a Leica TCS-NT confocal microscope. YFP-tagged fusion proteins were excited using the Ar laser line at 488 nm and detected at 500–530 nm (green channel). The images were assembled using the Leica confocal software LSC Lite version 2.61. For microscopic analysis of other reporter lines, plants were treated with Brz and BL as described previously [12] and were analysed with an Olympus Bx61 fluorescence microscope. For co-localization experiments, protoplasts were isolated from Arabidopsis mesophyll cell suspension culture and were transformed with 20 μg plasmid DNA (35S:CES S75A+S77A :YFP or 35S:COP1:CFP ) according to ref. 49 . The images were taken using an Olympus CLSM confocal microscope using defined settings for YFP and CFP. Protoplast transformation and transactivation assays For transactivation assays, protoplasts were isolated from bee1 bee3 haf triple mutants [13] and transiently transformed using a polyethyleneglycol-mediated transformation protocol as described previously [49] . Briefly, leaves of 4-week-old plants were cut into 0.5–1 mm strips with a razor blade and placed in freshly prepared enzyme solution (20 mM MES; pH 5.7, 1.5% (wt/vol) cellulase R10, 0.4% (wt/vol) macerozyme R10, 0.4 M mannitol, 10 mM CaCl 2 and 20 mM KCl). Leaf strips were vacuum infiltrated for 30 min using a desiccator and incubated in enzyme solution at room temperature in the dark for a further 3–4 h. The protoplast-containing enzyme solution was diluted with an equal volume of W5 buffer (2 mM MES; pH 5.7, 154 mM NaCl, 125 mM CaCl 2 and 5 mM KCl), filtered through Miracloth (Merck Biosciences, Nottingham, UK) and the flow-through was centrifuged at 100 g to obtain a pellet. The pellet was washed two times with W5 solution and the protoplasts were re-suspended in MMG solution (4 mM MES; pH 5.7, 0.4 M mannitol and15 mM MgCl 2 ) to obtain a final concentration of 2 × 10 5 ml –1 . 20 μg of DNA was used for each transformation and was diluted in a total volume of 20 μl to which 100 μl of protoplasts was gently added. Then, 120 μl of polyethyleneglycol solution was added slowly and mixed by tapping, and the mixture was incubated on ice for 30 min. In total, 440 μl W5 solution was added to dilute the mixture, mixed by inverting the tubes and centrifuged at 100 g for 2 min at room temperature. The supernatant was removed and the protoplasts were re-suspended in 200 μl of WI solution (4 mM MES; pH 5.7, 0.5 M mannitol and 20 mM KCl) and incubated overnight at room temperature. Luciferase assays were performed using a Dual-Luciferase Reporter Assay System (Promega, Madison, WI, USA) according to ref. 49 and utilizing a Lumat LB9501 luminometer (Berthold, Bad Wildbach, Germany) for signal quantification. In vitro SUMOylation assays and western blot analysis HIS-tagged SUMO modifiers and GST-tagged CES wild type and mutant proteins were purified using nickel (Carl Roth, Karlsruhe, Germany) and glutathione-sepharose beads (GE Healthcare) as recommended by the suppliers. In vitro SUMOylation assays were modified from ref. 50 . Briefly: 2 μg of protein substrates were incubated with 2 μg of recombinant SUM1 or SUM2, 1 μg SAE (Boston Biochem, Cambridge, MA, USA), 0.5 μg SCE (Boston Biochem) and 1 × SUMO buffer (20 mM Tris/HCl pH=7.5, 5 mM MgCl 2 ) in a total volume of 20 μl and in the presence of ATP. The reactions were incubated overnight at 30 °C and then stopped by adding 6 μl 4 × SDS sample buffer (200 mM Tris/HCl pH=6.8, 400 mM dithiothreitol (DTT), 80 g l −1 SDS, 400 g l −1 glycerol, 0.1 g l −1 bromophenol blue) and incubating at 95 °C for 5 min. The reaction products were separated on a 10% SDS gel and detected by western blot analysis. Membranes were probed with a polyclonal α-CES rabbit antibody (1:5,000 dilution) raised against a mixture of the peptides ARFEPYNYNNGHDPF and SVGTQPPNFSSTLPF corresponding to amino acids 2–16 and 209–223 of CES, respectively (generated by Eurogentec S.A., Seraing, Belgium). Alkaline phosphatase-conjugated goat α-rabbit IgG (Santa Cruz Biotechnology, CA, USA) was used as secondary antibody and was detected by enhanced chemiluminescence using CDP-Star reagent (GE Healthcare). For analysis of proteins in transgenic plant lines, 100 mg of tissue was ground to a fine powder and 300 μl of 1.33 × SDS sample buffer was added. The samples were heated at 95 °C for 5 min and 20 μl of protein extracts were separated by SDS-PAGE. Membranes were probed with a mouse α-GFP primary antibody (1:5,000 dilution) (Roche Diagnostics, Indianapolis, IN, USA). Alkaline phosphatase-conjugated goat α-mouse IgG (Sigma-Aldrich, Steinheim, Germany) was used as secondary antibody and was detected by enhanced chemiluminescence using CDP-Star reagent (GE Healthcare). Uncropped scans of western blots and CBB stained gels shown in the main manuscript are given in Supplementary Fig. 6 . Co-immunoprecipitation and chromatin-immunoprecipitation For co-immunoprecipitation experiments, Arabidopsis protoplasts were transformed with 35S:CES S75A+S77A -Myc (6) , were harvested and re-suspended in buffer A (50 mM Tris-HCl pH 7.4, 100 mM NaCl, 10% glycerol) supplemented with 0.2% Triton-100, 5 mM N -ethylmaleimide and 100 μM MG132. Following incubation on ice for 15 min, the samples were centrifuged for 10 min at 13,000 r.p.m. at 4 °C and the supernatants were divided into two parts to each of which 150 μl of protein A beads was added. After an incubation for 15 min at 4 °C (pre-clearing), the supernatants were transferred to fresh tubes and 2 μl of α-Myc (mouse) antibody was added to one of the tubes (the second was used as control). After another incubation step at 4 °C for 30 min, 150 μl of protein A beads were added to both tubes and incubated for further 30 min. The beads were washed twice with ice-cold buffer A, re-suspended in 1 × SDS loading buffer without DTT, incubated at 95 °C for 3 min and filtered with SpinPrep columns (Sigma). A total of 15 μl immuno-precipitated proteins were separated on a 10% SDS gel and immuno-detected with a rabbit α-SUMO antibody (1:3,000 dilution; Abcam, Cambridge, UK). Alkaline phosphatase-conjugated goat α-rabbit IgG (Sigma-Aldrich) was used as secondary antibody and detected by enhanced chemiluminescence using the CDP-Star reagent (GE Healthcare). Chromatin-immunoprecipitation experiments were performed as described previously [12] . In vitro kinase assays and mass spectrum analysis For in vitro kinase assays from plant extracts, inflorescence of Arabidopsis plants were harvested, ground to a fine powder in liquid nitrogen and total proteins were extracted in lacus buffer (25 mM Tris/HCl pH 7.8; 10 mM EGTA; 10 mM MgCl 2 ; 75 mM NaCl; 1 mM DTT; 1 mM NaF; 0.5 mM NaVO 3 ; 15 mM β-glycero-phosphate; 15 mM 4-nitophenyl-phosphate di-TRIS salt); 0.1% Tween 20; 0.5 mM PMSF; 5 μg ml −1 leupeptine and 5 μg ml −1 aprotinin). In total, 100 μg of total protein extract was used for incubation with 2 μg of protein substrate in the presence of 1 × kinase buffer (20 mM HEPES pH 7.4; 15 mM MgCl 2 ; 5 mM EGTA; 1 mM DTT) and [γ- 32 P]ATP in a total volume of 500 μl. The proteins were immuno-precipitated with GSH beads (GE Healthcare), washed with 1 × PBS containing 5 mM DDT. The product was subjected to SDS-PAGE. In vitro kinase assays with BIN2 and mass spectrometric analysis of BIN2-phosphorylated CES were performed as described previously [30] . For in vitro kinase assays with CDPKs, proteins were expressed in E. coli ER2566. Protein expression was induced by adding 1 mM isopropyl-β-D-thiogalactoside to exponentially growing cells followed by an incubation at 16 °C for 12 h. For protein extraction, E. coli cells were re-suspended in buffer B1 (20 mM HEPES pH 7.0, 1 M NaCl, 1 mM EDTA, 0.2 mM 2-mercaptoethanol) at 4 °C. Subsequently, the cell suspension was sonicated and the cell debris was afterwards removed by centrifugation at 16,000 g for 20 min at 4 °C. The supernatant was filtered through four layers of Miracloth (Calbiochem, La Jolla, CA, USA) and applied to a column packed with 2-ml chitin beads (New England Biolabs) equilibrated with buffer B1. The column was washed with 10-column volumes of buffer B1 and 2-column volumes of buffer B2 (20 mM HEPES pH 7.0, 500 mM NaCl, 1 mM EDTA, 0.2 mM 2-mercaptoethanol). To obtain the tag-free protein intein cleavage was induced by incubating the columns at 25 °C for 12 h. Proteins were then eluted in 4 ml of buffer B2. Subsequently, proteins were concentrated and transferred into kinase assay buffer (20 mM HEPES pH 7.5, 20 mM MgCl 2 , 1 mM DTT, 0.05% TWEEN 20, 50 μM CaCl 2 ) using Amicon Ultra centrifugal filters (Millipore, Bedford, MA, USA) with appropriate molecular weight cutoffs for the expressed kinases, according to the manufacturer’s instructions. For in vitro kinase assays with CDPKs, kinase reactions were performed in kinase assay buffer (20 mM HEPES pH 7.5, 20 mM MgCl 2 , 1 mM DTT, 0.05% (v/v) TWEEN 20, 50 μM CaCl 2 ) containing 0.1 μg μl −1 CDPKs and 2 μg μl −1 of the different CES variants. The reactions were started by adding first 50 μM cold ATP and second 20 nM active [γ- 32 P]ATP (6,000 Ci mmol −1 ; Perkin Elmer, Waltham, MA, USA) were incubated at 20 °C for 15 min and were then stopped by adding SDS-PAGE loading buffer. The reactions were incubated at 95 °C for 5 min, were separated by SDS-PAGE and stained with coomassie brilliant blue. To analyse the kinase reactions, the dried gel was exposed to a Storage Phosphoscreen (GE Healthcare), which was read out after 30 min by a Typhoon Trio Imager (GE Healthcare). Transcript analysis cDNA was synthesized from DNaseI-treated total RNA isolated from plant tissue using the RevertAid H minus first-strand cDNA synthesis kit (Thermo Fisher Scientific, St Leon-Rot, Germany). PCR reactions were performed using gene-specific primers that amplified 60–100-bp large fragments located in the 3′ parts of the genes investigated. GAPC2 was used as an internal template control. qPCR was performed with the Eppendorf Real-Time PCR System (Eppendorf, Wesseling-Berzdorf, Germany). Each reaction contained 10 μl 2 × PCR Master Mix (Promega), 4 pmol of each primer and 5 μl cDNA (prepared as described and diluted 1:10) in a total volume of 20 μl. Cycling was performed as recommended by the manufacturer (initial denaturation: 94 °C for 10 min; 40 cycles at 94 °C for 15 s and 60 °C for 1 min) and finally a melting curve was recorded. A dilution series of cloned cDNA was run under the same conditions and the results were used to plot a calibration curve, which served to calculate the transcript abundance in the samples. The relative expression levels were calculated from four replicates and normalization to GAPC2. Standard deviations were deduced from three biological repeats. How to cite this article: Khan, M. et al. Interplay between phosphorylation and SUMOylation events determines CESTA protein fate in brassinosteroid signalling. Nat. Commun. 5:4687 doi: 10.1038/ncomms5687 (2014).